Quantum interference of large organic molecules The wave nature of matter is a key ingredient of quantum physics and yet it defies our classical intuition. First proposed by Louis de Broglie a century ago, it has since been confirmed with a variety of particles from electrons up to molecules. Here we demonstrate new high-contrast quantum experiments with large and massive tailor-made organic molecules in a near-field interferometer. Our experiments prove the quantum wave nature and delocalization of compounds composed of up to 430 atoms, with a maximal size of up to 60 Å, masses up to m =6,910 AMU and de Broglie wavelengths down to λ dB = h/mv ≃ 1 pm. We show that even complex systems, with more than 1,000 internal degrees of freedom, can be prepared in quantum states that are sufficiently well isolated from their environment to avoid decoherence and to show almost perfect coherence. In many discussions on the foundations of physics, single-particle diffraction at a double slit [1] , [2] , [3] , [4] or grating [5] , [6] , [7] , [8] , [9] , [10] , [11] , [12] is regarded as a paradigmatic example for a highly non-classical feature of quantum mechanics, which has never been observed for objects of our macroscopic world. The quantum superposition principle has become of paramount importance also for the growing field of quantum information science [13] . Correspondingly, research in many laboratories around the world is focusing on our understanding of the role of decoherence for increasingly complex quantum systems and possible practical or truly fundamental limits to the observation of quantum dynamics [14] , [15] . Here we report on a new leap in quantum interference with large organic molecules. In contrast to earlier successful experiments with internal molecular wave packets, [16] our study focuses on the wave evolution in the centre of mass motion of the molecule as a whole, that is, pure de Broglie interference. We do this with compounds that have been customized to provide useful molecular beams at moderate temperatures [17] , [18] . 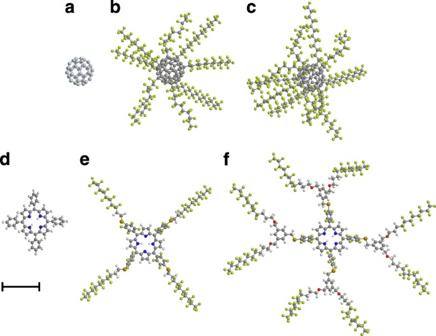Figure 1: Gallery of molecules used in our interference study. (a) The fullerene C60(m=720AMU, 60 atoms) serves as a size reference and for calibration purposes; (b) The perfluoroalkylated nanosphere PFNS8 (C60[C12F25]8,m=5,672AMU, 356 atoms) is a carbon cage with eight perfluoroalkyl chains. (c) PFNS10 (C60[C12F25]10,m=6,910AMU, 430 atoms) has ten side chains and is the most massive particle in the set. (d) A single tetraphenylporphyrin TPP (C44H30N4,m=614AMU, 78 atoms) is the basis for the two derivatives (e) TPPF84 (C84H26F84N4S4,m=2,814AMU, 202 atoms) and (f) TPPF152 (C168H94F152O8N4S4,m=5,310AMU, 430 atoms). In its unfolded configuration, the latter is the largest molecule in the set. Measured by the number of atoms, TPPF152 and PFNS10 are equally complex. All molecules are displayed to scale. The scale bar corresponds to 10 Å. Figure 1 compares the size of two perfluoroalkylated nanospheres, PFNS8 and PFNS10, with a single C 60 fullerene [19] and it relates a single tetraphenylporphyrin molecule (TPP) to its complex derivatives TPPF84 and TPPF152. 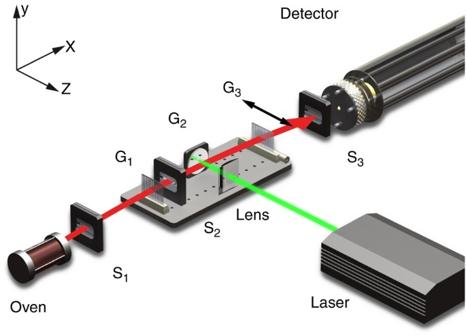Figure 2: Layout of the Kapitza-Dirac-Talbot-Lau (KDTL) interference experiment. The effusive source emits molecules that are velocity-selected by the three delimiters S1, S2and S3. The KDTL interferometer is composed of two SiNxgratings G1and G3, as well as the standing light wave G2. The optical dipole force grating imprints a phase modulationϕ(x)∝αopt·P/(v·wy) onto the matter wave. Hereαoptis the optical polarizability,Pthe laser power,vthe molecular velocity andwythe laser beam waist perpendicular to the molecular beam. The molecules are detected using electron impact ionization and quadrupole mass spectrometry. We demonstrate the wave nature of all these molecules in a three-grating near-field interferometer [20] , [21] of the Kapitza-Dirac-Talbot-Lau type [22] , [23] , as shown in Figure 2 . Figure 1: Gallery of molecules used in our interference study. ( a ) The fullerene C 60 ( m =720 AMU , 60 atoms) serves as a size reference and for calibration purposes; ( b ) The perfluoroalkylated nanosphere PFNS8 (C 60 [C 12 F 25 ] 8 , m =5,672 AMU , 356 atoms) is a carbon cage with eight perfluoroalkyl chains. ( c ) PFNS10 (C 60 [C 12 F 25 ] 10 , m =6,910 AMU , 430 atoms) has ten side chains and is the most massive particle in the set. ( d ) A single tetraphenylporphyrin TPP (C 44 H 30 N 4 , m =614 AMU , 78 atoms) is the basis for the two derivatives ( e ) TPPF84 (C 84 H 26 F 84 N 4 S 4 , m =2,814 AMU , 202 atoms) and ( f ) TPPF152 (C 168 H 94 F 152 O 8 N 4 S 4 , m =5,310 AMU , 430 atoms). In its unfolded configuration, the latter is the largest molecule in the set. Measured by the number of atoms, TPPF152 and PFNS10 are equally complex. All molecules are displayed to scale. The scale bar corresponds to 10 Å. Full size image Figure 2: Layout of the Kapitza-Dirac-Talbot-Lau (KDTL) interference experiment. The effusive source emits molecules that are velocity-selected by the three delimiters S 1 , S 2 and S 3 . The KDTL interferometer is composed of two SiN x gratings G 1 and G 3 , as well as the standing light wave G 2 . The optical dipole force grating imprints a phase modulation ϕ (x) ∝ α opt · P /( v · w y ) onto the matter wave. Here α opt is the optical polarizability, P the laser power, v the molecular velocity and w y the laser beam waist perpendicular to the molecular beam. The molecules are detected using electron impact ionization and quadrupole mass spectrometry. Full size image Experimental setup The particles are evaporated in a thermal source. Their velocity is selected using the gravitational free-fall through a sequence of three slits. The interferometer itself consists of three gratings G 1 , G 2 and G 3 in a vacuum chamber at a pressure of p <10 −8 mbar. The first grating is a SiN x membrane with 90-nm wide slits arranged with a periodicity of d =266 nm. Each slit of G 1 imposes a constraint onto the transverse molecular position that, following Heisenberg's uncertainty relation, leads to a momentum uncertainty. The latter turns into a growing delocalization and transverse coherence of the matter wave with increasing distance from G 1 . The second grating, G 2 , is a standing laser light wave with a wavelength of λ =532 nm. The interaction between the electric laser light field and the molecular optical polarizability creates a sinusoidal potential, which phase-modulates the incident matter waves. The distance between the first two gratings is chosen such that quantum interference leads to the formation of a periodic molecular density pattern 105 mm behind G 2 . This molecular nanostructure is sampled by scanning a second SiN x grating (G 3 , identical to G 1 ) across the molecular beam while counting the number of the transmitted particles in a quadrupole mass spectrometer (QMS). In extension to earlier experiments, we have added various technological refinements: the oven was adapted to liquid samples, a liquid-nitrogen-cooled chamber became essential to maintain the source pressure low, a new mass analyser allowed us to increase the detected molecular flux by a factor of four and many optimization cycles in the interferometer alignment were needed to meet all requirements for high-contrast experiments with very massive particles. 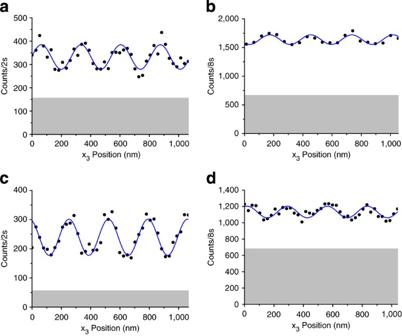Figure 3: Quantum interferograms of tailor-made large organic molecules. Quantum interference well beyond the classical expectations has been observed for all molecules in the set. In all panels, the black circles represent the experimental result, the blue line is a sinusoidal fit to the data and the shaded area indicates the detector dark rate. (a) The beam of perfluoroalkylated nanospheres, PFNS8, is characterized by a mean velocity ofv=63 m s−1with a full width ΔvFWHM=13 m s−1. The observed contrast ofVobs=49±6% is in good agreement with the expected quantum contrast ofVquant=51% and is clearly discernible from the classically expected visibility ofVclass<1%. The stated uncertainty is the standard deviation of the fit to the data. (b) For PFNS10, the signal was too weak to allow a precise velocity measurement and quantum calculation. The oven position for these particles, however, limits the molecular velocity tov<80 m s−1and therefore allows us to define an upper bound to the classical visibility. (c) For TPPF84, we measurev=95 m s−1with ΔvFWHM=34 m s−1. This results inVobs=33±3% withVquant=30% andVclass<1%. (d) The signal for TPPF152 is equally low compared with that of PFNS10. For this compound we findVobs=16±2%,Vquant=45% andVclass=1%. Observed interferograms We recorded quantum interferograms for all molecules of Figure 1 , as shown in Figure 3 . In all cases the measured fringe visibility V , that is, the amplitude of the sinusoidal modulation normalized to the mean of the signal, exceeds the maximally expected classical moiré fringe contrast by a significant multiple of the experimental uncertainty. This is best shown for TPPF84 and PFNS8, which reached the highest observed interference contrast in our high-mass experiments so far, with individual scans up to V obs =33% for TPPF84 ( m =2,814 AMU ) and V obs =49% for PFNS8 at a mass of m =5,672 AMU . In addition, we have observed a maximum contrast of V obs =17±4% for PFNS10 and V obs =16±2% for TPPF152 (see Figure 3 ), in which our classical model predicts V class =1%. This supports our claim of true quantum interference for all these complex molecules. Figure 3: Quantum interferograms of tailor-made large organic molecules. Quantum interference well beyond the classical expectations has been observed for all molecules in the set. In all panels, the black circles represent the experimental result, the blue line is a sinusoidal fit to the data and the shaded area indicates the detector dark rate. ( a ) The beam of perfluoroalkylated nanospheres, PFNS8, is characterized by a mean velocity of v =63 m s −1 with a full width Δ v FWHM =13 m s −1 . The observed contrast of V obs =49±6% is in good agreement with the expected quantum contrast of V quant =51% and is clearly discernible from the classically expected visibility of V class <1%. The stated uncertainty is the standard deviation of the fit to the data. ( b ) For PFNS10, the signal was too weak to allow a precise velocity measurement and quantum calculation. The oven position for these particles, however, limits the molecular velocity to v <80 m s −1 and therefore allows us to define an upper bound to the classical visibility. ( c ) For TPPF84, we measure v =95 m s −1 with Δ v FWHM =34 m s −1 . This results in V obs =33±3% with V quant =30% and V class <1%. ( d ) The signal for TPPF152 is equally low compared with that of PFNS10. For this compound we find V obs =16±2%, V quant =45% and V class =1%. Full size image The most massive molecules are also the slowest and therefore the most sensitive ones to external perturbations. In our particle set, these are PFNS10 and TPPF152, which, in addition, exhibited the smallest count rates and therefore the highest statistical fluctuations. To record the interferograms, we had to open the vertical beam delimiter S 2 and accept various imperfections: an increased velocity spread, a higher sensitivity to grating misalignments and also an averaging over intensity variations in the Gaussian-shaped diffraction laser beam G 2 . In addition, we had to enhance the QMS transmission efficiency at the expense of transmitting a broader mass range. The recorded signals associated with PFNS10 and TPPF152 covered a mass window of Δ m FWHM =500 AMU around their nominal masses. Although all samples were well characterized before the evaporation process, we can therefore not exclude some contamination with adducts or fragments in this high mass range. But even if there were a relative mass spread of 10%, this would only influence the wavelength distribution Δ λ dB / λ dB the same way as does the velocity spread. Owing to the inherent design of the Kapitza-Dirac-Talbot-Lau interferometer [22] , these experimental settings are still compatible with sizeable quantum interference, even under such adverse conditions. Comparison of theory and experiment The experimental values have to be compared with the theoretical predictions based on a classical and a quantum model [23] . 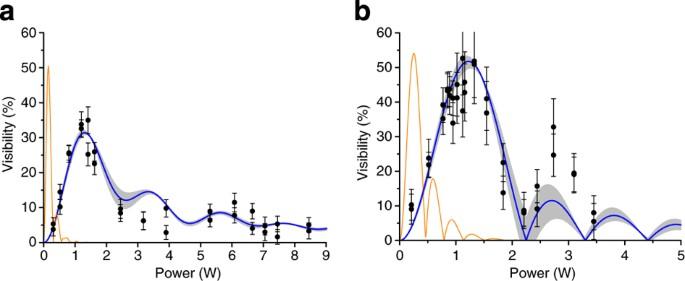Figure 4: Quantum interference visibility as a function of the diffracting laser power. The best distinction between quantum and classical behaviour is made by tracing the interference fringe visibility as a function of the laser power, which determines the phase imprinted by the second grating. Each of the two experimental runs per molecule is represented by full circles and the error bar provides the 68% confidence bound of the sinusoidal fit to the interference fringe. The thick solid line is the quantum fit in which the shaded region covers a variation of the mean molecular velocity by Δv=±2 m s−1. (a) The TPPF84 data are well reproduced by the quantum model (see text) and completely missed by the classical curve (thin line on the left). (b) The same holds for PFNS8. The following parameters were used for the models: TPPF84:v=95 m s−1±16%,α=200 Å3×4πɛ0(fit),σopt=10−21m−2,wx=34±3 μm andwy=500±50 μm. PFNS8:v=75 m s−1±10%,α=190 Å3×4πɛ0(fit),σopt=10−21m−2,wx=27±3 μm andwy=620±50 μm. The measured interference visibility is plotted as a function of the diffracting laser power P in Figure 4 for TPPF84 (4a) and PFNS8 (4b). Our data are in very good agreement with the full quantum calculation and in clear discrepancy with the classical prediction. The abscissa scaling of the V ( P ) curve is a good indicator for that. The quantum prediction mimics the classical curve qualitatively, but it is stretched in the laser power by a factor of about six (see Methods). Figure 4: Quantum interference visibility as a function of the diffracting laser power. The best distinction between quantum and classical behaviour is made by tracing the interference fringe visibility as a function of the laser power, which determines the phase imprinted by the second grating. Each of the two experimental runs per molecule is represented by full circles and the error bar provides the 68% confidence bound of the sinusoidal fit to the interference fringe. The thick solid line is the quantum fit in which the shaded region covers a variation of the mean molecular velocity by Δ v =±2 m s −1 . ( a ) The TPPF84 data are well reproduced by the quantum model (see text) and completely missed by the classical curve (thin line on the left). ( b ) The same holds for PFNS8. The following parameters were used for the models: TPPF84: v =95 m s −1 ±16%, α =200 Å 3 ×4πɛ 0 (fit), σ opt =10 −21 m −2 , w x =34±3 μm and w y =500±50 μm. PFNS8: v =75 m s −1 ±10%, α =190 Å 3 ×4πɛ 0 (fit), σ opt =10 −21 m −2 , w x =27±3 μm and w y =620±50 μm. Full size image The laser power can be calibrated with an accuracy of ±1% but the abscissa also scales in proportion to the optical molecular polarizability and inversely with the vertical laser waist. The theoretical curves of Figure 4 are plotted assuming α opt =200 Å 3 ×4πɛ 0 for TPPF84 and α opt =190 Å 3 ×4πɛ 0 for PFNS8. These numbers have to be compared with the static polarizabilities computed using Gaussian09 (ref. 24 ). These are α stat =155 Å 3 ×4πɛ 0 for TPPF84 and α stat =200 Å 3 ×4πɛ 0 for PFNS8. A variation in the polarizability changes the horizontal scale of the plot as does a different laser waist. Both are bound by a relative uncertainty of less than 30%. A classical explanation is therefore safely excluded as an explanation for the experiments. The quantitative agreement of the experimental and expected contrast is surprisingly good, given the high complexity of the particles. Various factors contribute to the remaining small discrepancies. The interference visibility is highly sensitive to apparatus vibrations, variations in the grating period on the level of 0.5 Å and a misalignment below 100 μrad in the grating roll angle. PFNS10 and TPPF152 contain 430 atoms covalently bound in one single particle. This is ∼ 350% more than that in all previous experiments [25] and it compares well with the number of atoms in small Bose–Einstein condensates [26] (BEC), which, of course, operate in a vastly different parameter regime: The molecular de Broglie wavelength λ dB is about six orders of magnitude smaller than that of ultracold atoms and the internal molecular temperature exceeds typical BEC values (T<1 μK) by about nine orders of magnitude. Although matter wave interference of BECs relies on the de Broglie wavelength of the individual atoms, our massive molecules always appear as single entities. One can find various definitions in the literature for what a true Schrödinger cat [27] should be and a number of intriguing experiments have reported the generation of photonic [28] or atomic cat-states [29] , [30] . In as far as the term designates the quantum superposition of two macroscopically distinct states of a highly complex object, the molecules in our new experimental series are among the fattest Schrödinger cats realized to date. Schrödinger reasoned whether it is possible to bring a cat into a superposition state of being 'dead' and 'alive'. In our experiment, the superposition consists of having all 430 atoms simultaneously 'in the left arm' and 'in the right arm' of our interferometer, that is, two possibilities that are macroscopically distinct. The path separation is about two orders of magnitude larger than the size of the molecules. Schrödinger's thought experiment originally also required the entanglement between a microscopic atom and the final state of the macroscopic cat. Such a mechanism is not needed to create the molecular superposition state in our experiment. Entanglement between a molecule and a microscopic probe particle does, however, occur in decoherence processes in which the quantum interaction with the environment reveals which-path information [14] , [15] and destroys the interference pattern. Collisions with residual gas molecules [31] , the emission of heat radiation [32] and the absorption of blackbody radiation are among the most important decoherence mechanisms for interferometry with massive particles. We estimate that they lead to a visibility reduction of less than 1% under the conditions of the present experimental arrangement, in spite of the high internal molecular temperatures and substantial dipole fluctuations. Specifically for PFNS8, a microscopically realistic account of the decoherence processes [31] , [32] predicts a visibility reduction of 10% only if the temperature of either the molecule or the radiation field exceeds 1,500 K, or if the residual nitrogen gas pressure exceeds 2×10 −7 mbar. In conclusion, our experiments reveal the quantum wave nature of tailor-made organic molecules in an unprecedented mass and size domain. They open a new window for quantum experiments with nanoparticles in a complexity class comparable to that of small proteins, and they demonstrate that it is feasible to create and maintain high quantum coherence with initially thermal systems consisting of more than 1,000 internal degrees of freedom. Chemical synthesis The porphyrin derivatives were synthesized by the attachment of a highly fluorous thiol to meso-tetra(pentafluorophenyl)porphyrin in a nucleophilic aromatic substitution reaction by applying a modified literature procedure [33] . To assemble TPPF84, the commercially available 1 H ,1 H ,2 H ,2 H -perfluorododecane-1-thiol as nucleophilic fluorous part was introduced to the porphyrin unit. The branched thiol building block for TPPF152 was synthesized in three reaction steps. A reaction sequence including mono-functionalization of tris(bromomethyl)benzene with a protected thiol, introduction of two fluorous ponytails and a final deprotection of the thiol functionality yielded the desired fluorous thiol suitable for the envisaged substitution reaction. All target structures were purified by column chromatography and characterized by nuclear magnetic resonance spectroscopy and mass spectrometry (Supplementory Methods). Differences between the classical and quantum predictions The functional dependence of the interference fringe visibility on the laser power is qualitatively similar in both a classical and a full quantum treatment. As observed from the treatment described in ref. 23 the abscissa scaling differs, however, by the factor ξ/sin(ξ) with ξ=π· L / L T , where L is the distance between two consecutive gratings and L T = d 2 / λ dB is the Talbot length. For the case of Figure 4 , we find ξ/sin(ξ) ≃ 5.9. The experimental data are in clear agreement with the quantum model. Equipment The diffracting laser beam is generated by a Coherent Verdi V18 laser at 532 nm. The QMS is an Extrel CMS with a rod diameter of 9.5 mm, operated at a radio frequency of 440 kHz. The SiN x gratings in G 1 and G 3 were made by Dr Tim Savas, nm 2 LLC & MIT Cambridge. How to cite this article: Gerlich, S. et al . Quantum interference of large organic molecules. Nat. Commun. 2:263 doi: 10.1038/ncomms1263 (2011).